Optical solitons in graded-index multimode fibres Solitons are non-dispersing localized waves that occur in diverse physical settings, including liquids, optical fibres, plasmas and condensed matter. They attract interest owing to their particle-like nature and are useful for applications such as in telecommunications. A variety of optical solitons have been observed, but versions that involve both spatial and temporal degrees of freedom are rare. Optical fibres designed to support multiple transverse modes offer opportunities to study wave propagation in a setting that is intermediate between single-mode fibre and free-space propagation. Here we report the observation of optical solitons and soliton self-frequency shifting in graded-index multimode fibre. These wave packets can be modelled as multicomponent solitons, or as solitons of the Gross–Pitaevskii equation. Solitons in graded-index fibres should enable increased data rates in low-cost telecommunications systems, are pertinent to space-division multiplexing, and can offer a new route to mode-area scaling for high-power lasers and transmission. Solitons are localized waves that arise from the interplay of linear and nonlinear processes that individually would cause the wave to decay. They occur in numerous physical settings, including liquids [1] , [2] , optical fibres [3] , plasmas [4] and condensed matter [5] , [6] . Temporal solitons that form in single-mode optical fibre [7] , [3] are perhaps the quintessential example, and they have had major influence on telecommunications. The potential impact of soliton formation in multimode fibre was appreciated by early workers [8] , [9] , [10] . More recently, multimode fibre has been considered theoretically as an environment that could support spatiotemporal solitons [11] , [12] , or light bullets, which attract interest owing to their particle-like nature and potential for all-optical switching [13] , [14] , [15] , [16] . Perhaps surprisingly, no experiments have been reported despite the theoretical progress. Optical pulse propagation in a multimode fibre involves an intricate mix of spatiotemporal phenomena coupled fundamentally by nonlinearity and practically by waveguide imperfections. Modelling of the pulse propagation [8] , [9] , [10] , [17] , [18] is difficult, and multiple approaches have been taken. These include rewriting the coupled modes in terms of principal modes [19] , [20] , [21] , variational solution of a nonlinear wave equation [11] , [12] , [22] , and analysis of optical-wave thermalization and condensation [23] . From a modal perspective, soliton formation requires nonlinear coupling between the modes to cancel the effects of modal dispersion [8] , [9] , [10] . Such multicomponent or vector solitons have been studied in several contexts [24] , [25] , [26] . There is only one prior report of spatiotemporal vector solitons [14] , where the two components were different colours. Alternatively, nonlinear pulse pulse propagation in a multimode waveguide can be analyzed with a three-dimensional Gross–Pitaevskii equation [27] , which is widely used to model Bose-Einstein condensates. The soliton solutions simultaneously balance nonlinearity with diffraction, dispersion and a spatial harmonic potential. In addition to its intrinsic scientific interest, the formation of solitons in graded-index (GRIN) fibre will be relevant to applications. Owing to their low cost and ease of alignment, multimode fibres are widely used in high-speed local area networks [28] . The maximum data rate is limited by intersymbol interference that arises from modal dispersion. A new pulse propagation technique that can retain the simplicity of multimode systems while avoiding modal dispersion should be beneficial to low-cost, high-speed systems. As systems approach the Shannon limit for information transmission, interest in exploiting multiple spatial channels [29] , [30] , [31] , which could be transverse modes, has grown. Whether used to minimize cross-talk in neighbouring modes or to determine nonlinear limits to such approaches, soliton formation will be a factor in the design of such technologies. Finally, there is a growing need for large-mode-area fibres for the generation and transmission of pulses with ever-higher peak powers [32] . Soliton transmission through large-core GRIN fibres could have a major role in these applications. In this article, we describe theoretical and experimental observations of optical solitons and soliton self-frequency shifting in GRIN multimode fibre. Remarkably, the stable solutions of the coupled-mode equations and the Gross–Pitaevskii equation are equivalent. Implications of the results for telecommunication, space-division multiplexing and high-power laser and transmission systems are discussed. Coupled-mode analysis The most-complete theoretical model is based on coupled modes of the electromagnetic field [17] , [18] . The complex electric field can be decomposed into a sum of spatial functions for the modes, F p ( ρ , φ , ω ), multiplied by the evolving envelopes, A p ( z , ω ): To simplify the problem, we consider only the radially symmetric modes (written explicitly in Supplementary Note 1 ), which are relevant to our experiments. The normalized modes, F p ( ρ , ω ), and corresponding propagation constants, β p ( ω ), can be written as [18] where L p is a Laguerre polynomial, k = ωn 0 / c , Δ is the index difference between the centre and the cladding of the fibre, R is the fibre core radius, and w 0 =(2 R 2 / k 2 Δ) 1/4 is the fundamental mode size. By neglecting higher-order dispersive and nonlinear effects, the equations can then be written as where ( ) is the difference between the p th and the fundamental mode of the first (second) coefficient in the Taylor expansion of β p about ω 0 . β 2 corresponds to the material group-velocity dispersion, γ = ω 0 n 2 / c is the nonlinear coefficient, and η plnm are the nonlinear coupling coefficients (defined explicitly in Supplementary Note 1 ). The equations are solved numerically for a variety of input fields launched into 100 m of a standard GRIN fibre (parameters in Methods), to correspond to experiments described below. The number of modes, and hence equations, required to account for the pulse propagation depends on the modes that are initially seeded. For the cases studied here, the GRIN fibre is seeded by the output of a standard single-mode fibre and >99.9% of the energy is accounted for with only the 3 lowest order symmetric modes. In linear propagation, the modes separate in time owing to their different group velocities and the pulse duration in each mode increases because of material dispersion ( Fig. 1 ). The beam waist oscillates with period until the pulses separate temporally, after which the oscillation ceases and the spatial evolution is essentially that of the fundamental mode. At higher powers, nonlinearity balances the material dispersion, mode-coupling counteracts the group-velocity mismatch, and a multicomponent soliton forms. In other words, the duration and temporal location of light energy in each mode are locked, and remain unchanged with propagation. While the existence of solitons in multimode systems was suggested based on analytical arguments [8] , [9] , [10] , this is the first demonstration that multicomponent solitons are even theoretically stable in a complete numerical model of the coupled modes. The result of launching a 300-fs, ~0.5-nJ pulse is shown in Fig. 2 , for example. The three modes ( Fig. 2a ) overlap in time ( Fig. 2b ), with the group delay equal to an energy-weighted average of the modal delays. The spectra of the individual modes shift to have the same group-velocity, with the higher-order modes blue-shifted ( Fig. 2c ). The structured spectra result from radiation of energy from each mode as the soliton forms. Similar structure appears when solitons form in single-mode fibre ( Supplementary Fig. S1 ). The space-time profile is nearly symmetric ( Fig. 3a ), with a sech 2 temporal intensity profile ( Fig. 3b ) and a Gaussian spatial profile ( Fig. 3c ). The mode-field diameter (MFD) averaged over the pulse ( Fig. 3d ) oscillates around the fundamental mode size (2w 0 ) with a period equal to that of low-intensity light. The full-width at half-maximum pulse duration averaged over the beam ( Fig. 3e ) quickly converges to a steady solution that is ~100 times shorter than the output pulse duration would be due to group-velocity dispersion alone. 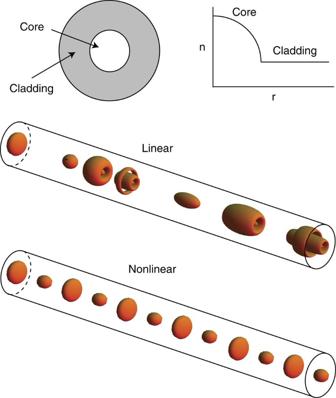Figure 1: Soliton formation in GRIN fiber. Top: Schematic of the core and cladding of the fiber and the relative index as a function of radius. Middle: In linear propagation, the spatial modes separate in time, and individually increase in duration. Bottom: Propagation of the soliton. Figure 1: Soliton formation in GRIN fiber. Top: Schematic of the core and cladding of the fiber and the relative index as a function of radius. Middle: In linear propagation, the spatial modes separate in time, and individually increase in duration. Bottom: Propagation of the soliton. 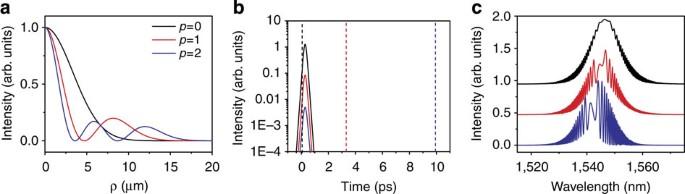Figure 2: Multicomponent soliton. (a) The three spatial modes and the corresponding (b) temporal pulse profiles and (c) normalized spectra. The dotted lines correspond to the location of the pulse centre after linear pulse propagation (without nonlinear attraction between modes). arb. unit, arbitrary unit. Full size image Figure 2: Multicomponent soliton. ( a ) The three spatial modes and the corresponding ( b ) temporal pulse profiles and ( c ) normalized spectra. The dotted lines correspond to the location of the pulse centre after linear pulse propagation (without nonlinear attraction between modes). arb. unit, arbitrary unit. 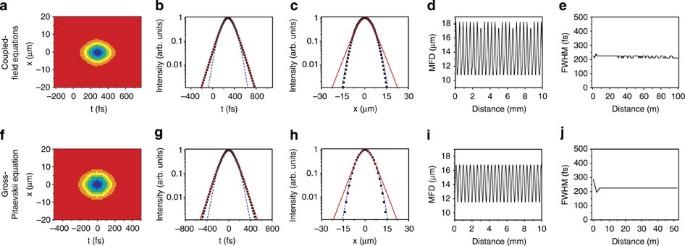Figure 3: Simulation results. Numerical solution of the coupled-field equations (a–e) and the Gross–Pitaevskii equation (f–j). (a) Space-time intensity plot, (b) pulse-averaged over space and (c) beam-averaged over time (symbols) with a hyperbolic secant squared (solid line) and Gaussian (dashed line) fits, evolution of the (d) spatial MFD averaged over the pulse and of the (e) full-width at half-maximum pulse duration averaged over the beam from the coupled-field equations and (f–j) the corresponding plots for the Gross–Pitaevskii equation. arb. unit, arbitrary unit. Full size image Figure 3: Simulation results. Numerical solution of the coupled-field equations ( a – e ) and the Gross–Pitaevskii equation ( f – j ). ( a ) Space-time intensity plot, ( b ) pulse-averaged over space and ( c ) beam-averaged over time (symbols) with a hyperbolic secant squared (solid line) and Gaussian (dashed line) fits, evolution of the ( d ) spatial MFD averaged over the pulse and of the ( e ) full-width at half-maximum pulse duration averaged over the beam from the coupled-field equations and ( f – j ) the corresponding plots for the Gross–Pitaevskii equation. arb. unit, arbitrary unit. Full size image Single-field analysis Alternatively, the system can be analyzed with a nonlinear wave equation for the total field. Standard procedures are used to reduce the Maxwell equations to a single wave equation. By employing the paraxial and slowly varying envelope approximations, a Gross–Pitaevskii equation is obtained [11] , [12] : where A is the slowly varying envelope at centre frequency ω 0 , , and t is time in a reference frame moving at the group-velocity of the pulse. The paraxial approximation does neglect the variation of group velocities among the modes. The approximation is justified in light of the solution to the coupled-field equations, which shows the modes aligning to a common group-velocity. To reach manageable computational times, we reduce the system to the two-dimensional case with y =0 as in Raghavan and Agrawal [12] . The solution quickly converges and simulations are stopped after 52 m of propagation (which requires 20 days of computation). Remarkably, the soliton solution is nearly identical to that found with the coupled-mode equations ( Fig. 3 ), except for a slight decrease in the amplitude of the spatial oscillation ( Fig. 3i ). The identification of terms in equation 4 with specific physical processes provides insight, but exact analytic solutions are not known. An approximate analytic solution is obtained by making the variational approximation with the trial function where is the energy, τ is the pulse duration, w 0 is the beam width, θ and α are chirp parameters, and φ is an arbitrary phase [33] , [12] , [11] . If the quantity is much less than one, a stable fixed point to the equations of motion is given by For typical fibre parameters =2 × 10 −4 , so the approximation is excellent. The fixed point is thus the fundamental mode of the GRIN fibre with a temporal profile that corresponds to the soliton with that beam size. Experiments The theoretical results suggest that the required pulse energy at 1,550 nm can be reached with readily designed Er-doped fibre lasers. Experiments were performed with a source that generates ~300-fs pulses (red lines in Fig. 4a and b ) with energy up to ~3 nJ. The initial spatial profile is the fundamental mode of an ordinary single-mode fibre with MFD of 11.5 μm ( Fig. 4c ). With these parameters, 100 m of GRIN fibre comprises ~100 dispersion lengths (that is, in linear propagation the pulse will broaden about 100 times), ~400 nonlinear lengths, and ~1,000,000 diffraction lengths ( Supplementary Note 2 ). For energies below 0.3 nJ the pulse disperses, and it is difficult to measure the autocorrelation of the output pulse. Results of launching a 0.5-nJ pulse illustrate soliton formation ( Fig. 4 ). After propagation through the fibre, the pulse is compressed temporally ( Fig. 4a ) and the spectrum becomes structured ( Fig. 4b ). The MFD at the end of the GRIN fibre is 17.9 μm ( Fig. 4d ). At higher energies, the output pulse duration decreases, and the spectrum broadens and red-shifts ( Fig. 5a ), in a manner immediately reminiscent of soliton self-frequency shifting [34] . 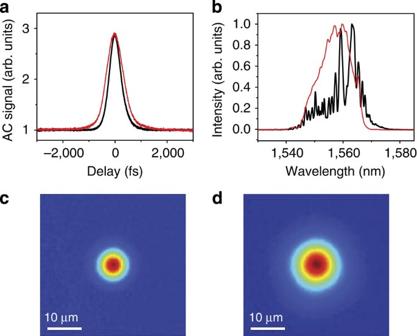Figure 4: Soliton formation with 0.5-nJ pulse energy. (a) Autocorrelation trace of the pulse and (b) spectrum before (red) and after (black) the GRIN fiber and beam profile (c) before and (d) after the GRIN fiber. arb. unit, arbitrary unit. Figure 4: Soliton formation with 0.5-nJ pulse energy. ( a ) Autocorrelation trace of the pulse and ( b ) spectrum before (red) and after (black) the GRIN fiber and beam profile ( c ) before and ( d ) after the GRIN fiber. arb. unit, arbitrary unit. 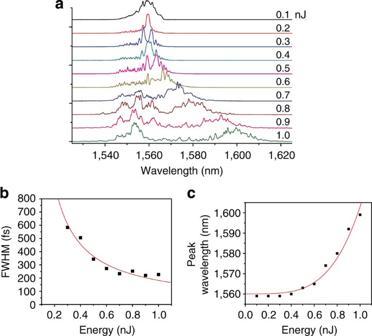Figure 5: Experimental trends with pulse energy. (a) Output spectra for indicated pulses energies. (b) Measured pulse duration versus energy (symbols) and fit to equation 6. (c) Measured peak wavelength versus pulse energy (symbols) and fit to equation 7. Full size image Figure 5: Experimental trends with pulse energy. ( a ) Output spectra for indicated pulses energies. ( b ) Measured pulse duration versus energy (symbols) and fit to equation 6. ( c ) Measured peak wavelength versus pulse energy (symbols) and fit to equation 7. Full size image We can conveniently analyze the experimental results using the results of the variational approach. The dependence of pulse duration on pulse energy is predicted well by the fixed point ( Fig. 5b ): the best fit is obtained with a MFD of 17.4 μm, which is close to the measured value of 17.9 μm. For the spectral shift we apply the results of standard soliton perturbation theory. The wavelength shift is inversely proportional to the fourth power of the pulse duration [34] : Here z is distance and T R is related to the slope of the Raman gain spectrum. The pulse duration is inversely proportional to the energy, so the wavelength shift should be proportional to the fourth power of the energy. Indeed this is the case ( Fig. 5c ): the best fit is obtained with T R =2.6 fs, which is close to the accepted value of 3 fs for silica fibre. The spatial and temporal degrees of freedom are coupled through the Kerr nonlinearity in a multimode waveguide. The picture that emerges from the theoretical and experimental results presented above is that a three-component soliton forms with nonlinear pulse propagation. That is, the process that is responsible for compensation of group-velocity dispersion in time also compensates for the separation of the different spatial modes (modal dispersion). The spatial evolution of the solitons in GRIN fibre has a significant linear contribution, as expected with a waveguide. However, the system differs significantly from a single-mode waveguide because the spatial dimensions have the freedom to have a major role. Therefore, it is surprising that, on average (ignoring spatial oscillations), the resulting solutions are equivalent to single-mode solitons propagating in the fundamental mode of the fibre. This is noteworthy considering that the system includes multiple modes (equation 3), and is modelled by a three-dimensional Gross–Pitaevskii equation (equation 4). Experimentally, measurements of the beam propagation on a sub-millimeter length scale will be valuable to confirm the presence of multiple transverse modes, but we are unable to make such measurements with adequate accuracy. While the analyses presented above clearly account well for the experiments, we cannot absolutely rule out an alternative explanation. Although the models would become quite complex, Raman scattering could be incorporated directly, rather than treated as a perturbation. In such a model, the interplay of linear mode-coupling (which distributes energy uniformly among modes) and Raman scattering could result in energy being ‘siphoned’ into the fundamental mode of the fibre [35] , [36] , [37] . The occurrence of this process would be noteworthy in its own right. We hope that the results presented here stimulate efforts to address this intriguing spatiotemporal problem. Regardless of the final theoretical interpretation, the observation of optical solitons and soliton self-frequency shifting in a GRIN waveguide has implications for a variety of scientific and technological issues. GRIN media offer a stable and convenient setting for the study of spatiotemporal wave propagation, with solutions that also pertain to Bose-Einstein condensates. Soliton transmission in multimode fibres relaxes the stringent coupling requirements for single-mode systems, and thereby could reduce the cost of high-data-rate telecommunication systems [28] . GRIN solitons will be pertinent to current efforts to reach the Shannon limit [38] through space-division multiplexing [29] , [30] , [31] . In such systems, cross-talk can be minimized by utilizing modes that do not overlap spatially as channels. Finally, the linear scaling of soliton energy and power with core diameter will benefit applications in high-power lasers and pulse transmission [32] . For example, commercially available GRIN fibre with 1-mm core diameter will allow transmission of 100-kW solitons. Coupled-mode analysis For the coupled equation simulations, λ 0 =1550, nm, E =0.5 nJ, n 2 =3.2 × 10 −20 m 2 W −1 , n 0 =1.444, β 2 =−281 fs 2 cm −1 , Δ=0.029, and R =31.25 μm. An overlap-integral calculation with a 10-μm Gaussian input reveals that >99.9% of the energy is accounted for with three modes (92.22% in p =0, 7.17% in p =1 and 0.56% in p =2). In linear propagation, the pulse in the p =1 mode moves away from the pulse in the fundamental mode at a rate of 33 fs m −1 (99 fs m −1 for p =2). Single-field analysis We use a split-step Fourier-transform method to numerically solve equation 4. With 1,024 points in time and 512 in space, and a 100-μm step in the propagation direction, simulation of pulse propagation through 52 m of fibre requires 20 days of computation using four cores on an Intel i7 computer. The parameters used for the simulations are the same as those for the coupled system, with an effective length of 11.8 μm for the y dimension. Experimental set-up Experiments were performed at 1550-nm wavelength where the group-velocity dispersion of fused silica is anomalous. An Erbium-doped fibre oscillator (11 MHz repetition rate) operating in the normal-dispersion regime produces ~300-fs pulses with ~1-nJ pulse energy. The oscillator is followed by 80 m of normal-dispersion fibre stretcher, a single-mode amplifier, and a transmission grating compressor in a standard chirped-pulse amplifier configuration. The output is aligned into a SMF-28 fibre pigtailed collimator of 50-cm length, which allows for near ideal seeding conditions ( Supplementary Fig. S2 ) when it is spliced directly to the GRIN fibre (Thorlabs GIF625). After all losses due to the grating compressor and coupling into the collimator, this set-up allows for up to ~3 nJ at a dechirped duration of ~300 fs. Experimental measurements The pulse is directly measured with a two-photon intensity autocorrelator, the spectrum is measured with a grating spectrometer with 0.4-nm resolution, and the beam is measured with an InGaAs camera with a 111 × beam expander to fill the detector array. The MFD is measured by averaging the widths of a Gaussian fit of the x and y cross-sections at the centre of the beam. The pulse duration as a function of energy for the pulses after the GRIN fibre are measured by taking the full-width at half-maximum duration of an intensity autocorrelation and dividing by the correlation factor for a sech 2 intensity profile (1.543). How to cite this article: Renninger W.H. et al. Optical solitons in graded-index multimode fibres. Nat. Commun. 4:1719 doi: 10.1038/ncomms2739 (2013).